Malaria oocysts require circumsporozoite protein to evade mosquito immunity Malaria parasites are less vulnerable to mosquito immune responses once ookinetes transform into oocysts, facilitating parasite development in the mosquito. However, the underlying mechanisms of oocyst resistance to mosquito defenses remain unclear. Here, we show that circumsporozoite protein (CSP) is required for rodent malaria oocysts to avoid mosquito defenses. Mosquito infection with CSP mut parasites (mutation in the CSP pexel I/II domains) induces nicotinamide adenine dinucleotide phosphate (NADPH) oxidase 5 (NOX5)-mediated hemocyte nitration, thus activating Toll pathway and melanization of mature oocysts, upregulating hemocyte TEP1 expression, and causing defects in the release of sporozoites from oocysts. The pre-infection of mosquitoes with the CSP mut parasites reduces the burden of infection when re-challenged with CSP wt parasites by inducing hemocyte nitration. Thus, we demonstrate why oocysts are invisible to mosquito immunity and reveal an unknown role of CSP in the immune evasion of oocysts, indicating it as a potential target to block malaria transmission. Malaria, one of the most devastating diseases worldwide, is transmitted through the bite of a Plasmodium -infected mosquito. The development of malaria parasites in the Anopheles mosquito begins with the transformation of ingested gametocytes into gametes in the midgut. Microgametes fertilize macrogametes to generate zygotes, which are then activated to form motile ookinetes that transverse the peritrophic matrix and midgut epithelium. Underneath the midgut epithelium, zygotes transform into oocysts that generate thousands of sporozoites, which are then released into the mosquito hemolymph, and finally invade the salivary glands. After feeding on a rodent host, blood taken into the mosquito midgut triggers the secretion of peroxidase/oxidase that catalyzes the crosslinking of proteins in the mucin layer of the mosquito midgut, which prevents gut bacteria and Plasmodium parasites from coming into direct contact with the midgut epithelium and eliciting an immune response [1] . However, a robust immune response is believed to be initiated when ookinetes begin to penetrate midgut epithelial cells. Ookinete invasion first induces the expression of nitric oxide synthase (NOS) and the production of nitric oxide (NO) in midgut epithelial cells [2] and then upregulates the expression of both heme peroxidase (HPX2) and nicotinamide adenine dinucleotide phosphate (NADPH) oxidase 5 (NOX5). These oxidases, together with NOS, mediate epithelial nitration, which make ookinetes visible to the mosquito immune system [3] , [4] . The nitrated midgut epithelial cells trigger the associated hemocytes to release hemocyte-derived microvesicles, which then activates complement-like thioester containing protein 1 (TEP1) to lyse parasites [5] . In addition to eliciting a local immune response, ookinetes can trigger systemic mosquito immune responses by inducing the midgut epithelium to secrete prostaglandin [6] , which in turn, stimulates the production of hemocyte differentiation factor, which induces hemocyte differentiation and establishes immune memory against the parasites [7] , [8] . To facilitate their development in mosquitoes, ookinetes have developed strategies to escape mosquito immune responses. For instance, Pfs47 , a Plasmodium falciparum gene, has been shown to suppress the mosquito immune system, allowing the parasite to infect Anopheles gambiae [9] , [10] . Pfs47 disrupts JNK-mediated apoptosis and suppresses nitration of ookinete-invaded midgut cells, which are critical for activating the complement-like system [4] , [11] . The mosquito immune response can also limit the development of oocysts through the generation of NOS dependent on a signal transducer and activator of transcription (STAT) [12] , hemocyte differentiation induced by lipopolysaccharide-induced TNFα transcription factor-like transcription factor 3 [12] , [13] , and pro-phenoloxidase (PPO) produced by hemocytes [14] , [15] . However, as compared to ookinetes, oocysts are less susceptible to the effects of mosquito immune defense, which facilitates their survival and development in mosquito hosts [16] . In addition, the lowest number of parasites in mosquitoes occurs at the oocyst stage, strongly suggesting that this stage is the most vulnerable for the disruption of malaria transmission [16] . Therefore, understanding oocyst immune evasion strategies could help toward designing strategies to block malaria transmission [16] . In this work, we find that a mutation of the circumsporozoite protein (CSP) pexel I/II domain significantly alters the conformation of this protein, which make the parasites visible to the mosquito immune system, leading to the nitration of hemocytes, activation of the Toll pathway, and the release of TEP1. As a result, the release of CSP mut (CSP pexel I/II domain mutant parasite) sporozoites is greatly impaired due to TEP1-mediated melanization of mature oocysts. Thus, we reveal an unknown role of CSP in evading mosquito immune responses and suggest CSP as a potential target to block malaria transmission. The release of sporozoites from CSP mut oocyst in mosquitoes is greatly impaired The pexel I/II domain of CSP has been demonstrated to mediate its translocation from the parasitophorous vacuole into the cytoplasm of hepatocytes [17] ; however, whether this domain influences the development of malaria parasites in mosquitoes is still unknown. A recombinant malaria parasite of rodents, Plasmodium yoelii 265 BY CSP mut , was successfully generated by replacing the wild-type CSP with a CSP pexel I/II mutant using CRISPR-Cas9 technology (Fig. 1a , and Supplementary Fig. 1 ). The first, third, and fifth amino acids of pexel I (RNLNE) and pexel II (RLLGD) in wild-type CSP presented mutations from R, L, E and R, L, D to A, as previously reported [18] . Both the parasitemia and gametocytemia of mice infected with P. yoelii CSP mut were comparable to those of mice infected with the wild-type parasite ( P. yoelii CSP wt ), indicating that the CSP pexel I/II mutation had no effect on the development of either the asexual or sexual blood stages of the malaria parasite (Fig. 1b, c ). In addition, both the number and size of CSP mut oocysts were comparable to those of CSP wt parasites at the indicated time points in mosquitoes (Fig. 1d, e ). Although a few sporozoites were observed in the hemolymph, none were found in the salivary glands of mosquitoes infected with P. yoelii CSP mut (Fig. 1f, g ). We also successfully constructed a P. berghei CSP mut mutant [19] , and similar results were obtained (Fig. 1h, i ), implying that there was no species-specific effect on parasite development in mosquitoes when the CSP pexel I/II domain was mutated. Thus, our results strongly suggest that the release of sporozoites from CSP mut oocysts was significantly impaired. Fig. 1: Release of sporozoites from CSP mut oocyst in mosquitoes is greatly impaired. a Schematic representing the construction of the recombinant Plasmodium yoelii CSP mut parasite using CRISPR-Cas9. The amino acids of pexel I (RNLNE) and pexel II (RLLGD) in wild-type CSP were mutated into ANANA and ALAGA, respectively. Both the parasitemia ( b ) and gametocytemia ( c ) of mice ( n = 15) infected with the CSP wt or CSP mut parasites were compared at the indicated time points. The average number of oocysts ( d ) in mosquitoes ( n = 81) at day 7, and the average diameter of oocysts ( e ) under ×400 field in mosquitoes ( n = 40) at the indicated time points after feeding on CSP wt or CSP mut -infected mice. The average number of salivary gland sporozoites ( f ) in mosquitoes ( n = 90), and hemolymph sporozoites ( g ) in mosquitoes ( n = 60) infected with P. yoelii CSP wt or CSP mut parasites at the indicated time points were recorded. The average number of salivary gland sporozoites ( h ) in mosquitoes ( n = 90), and hemolymph sporozoites ( i ) in mosquitoes ( n = 60) infected with P. berghei CSP wt or CSP mut parasites at the indicated time points. For box-plot diagram ( d ): middle line represents median; boxes extend from the 25th to 75th percentiles. The whiskers mark the 10th and 90th percentiles. c , d A two-sided Student’s t -test was used for the statistical analysis. f – i A two-sided Mann–Whitney U test was used for the statistical analysis. The data were presented as the means ± SD; ns, no significance; p -values were shown. The data were combined based on three independent experiments ( b – i ). Source data are provided as a Source Data file. Full size image TEP1-mediated oocyst melanization contributes to the developmental arrest of mutant parasites To elucidate the mechanism underlying the developmental arrest, the development of P. yoelii CSP mut oocysts was investigated in detail. On day 9 post infection (PI), we found that melanization of mature CSP mut oocysts began, but with different amounts of black dots deposited inside the oocyst capsule on day 12 PI (Fig. 2a ). Under electronic microscopy, some mature CSP mut oocysts generated thousands of sporozoites with normal morphology, but many sporozoites were found to be vacuolated and partially melanized at day 11 PI. This was not observed for the matured CSP wt oocysts (Fig. 2b ). In addition, the percentage of the melanized CSP mut oocysts increased from an average of 28.2% on day 9, to 49.3% on day 12, and 73.2% on day 15 PI. No melanized oocysts were observed in CSP wt -infected mosquitoes at any of the time points (Fig. 2c ). To confirm the decrease in the number of released sporozoites from melanized mutant oocysts, midguts from both CSP wt and CSP mut parasite-infected mosquitoes were isolated on day 10 PI, incubated in vitro, and their capacity to release sporozoites was then compared. Mature CSP mut oocysts released considerably fewer sporozoites than mature CSP wt oocysts when incubated for longer than 2 h (Fig. 2d ). Thus, the melanization of mature oocysts was closely associated with the impaired release of sporozoites from CSP mut oocysts. Fig. 2: Parasite development arrest largely depends on TEP1-mediated mature CSP mut oocyst melanization. a Representative image of melanized Plasmodium yoelii CSP mut in mosquitoes under a light microscope on day 12 after a blood meal; scale bar 50 μm. b Representative electron micrograph of vacuolized or melanized sporozoites (white arrows) from P. yoelii CSP wt and CSP mut oocysts at day 11; scale bar 1 μm. c Statistical analysis between the percentage of melanized mature P. yoelii CSP wt and CSP mut oocysts in mosquitoes ( n = 45) at the indicated time points post blood feeding. d Average number of sporozoites released from P. yoelii CSP wt and CSP mut oocysts in mosquitoes ( n = 60) at indicated incubation times in vitro. e mRNA expression level of TEP1 in mosquitoes ( n = 15) infected with P. yoelii CSP wt and CSP mut at the indicated time points post blood feeding determined using real-time PCR. f TEP1 activation (100 kD band) in hemocytes from mosquitoes ( n = 40) infected with P. yoelii CSP wt and CSP mut parasites detected using western blot; S7 protein was used as an internal control (left). Pooled data was quantified and analyzed (right). g Representative image of TEP1 binding to P. yoelii CSP wt and CSP mut oocysts at day 7 PI stained with anti-CSP repeat and anti-TEP1 (left), and the percentage of oocysts from P. yoelii CSP wt or CSP mut parasite-infected mosquitoes ( n = 30) bound with TEP1 was statistically analyzed (right); scale bar 10 μm. Percentage of melanized mature oocysts ( h ) in P. yoelii CSP mut parasite-infected mosquitoes ( n = 60) at day 12 PI, and average number of hemolymph sporozoites ( i ) in mosquitoes ( n = 60) infected with CSP mut parasites at the indicated time points compared following TEP1 knockdown. d – f A two-sided Student’s t -test was used for the statistical analysis. c , g – i A two-sided Mann–Whitney U test was used for the statistical analysis. The data were presented as the means ± SD; ns, no significance; p -values were shown. The data were combined based on three independent experiments ( c – i ) or two independent experiments ( b ). Source data are provided as a Source Data file. Full size image In mosquitoes, melanization characterized by the synthesis and deposition of melanin was the response to remove dead parasites. Since TEP1 plays an important role in the killing of malaria parasites [20] , [21] , [22] , [23] , [24] , we investigated whether TEP1 was involved in the melanization of CSP mut oocysts. Both the expression and activation of TEP1 were evaluated in mosquitoes infected with CSP mut and CSP wt parasites. TEP1 mRNA levels were significantly upregulated in mosquitoes infected with the mutant parasites at day 5 PI, as compared to that observed for the CSP wt infection (Fig. 2e ). Consistently, more TEP1 was activated in the hemolymph of mosquitoes infected with mutant parasites than those infected with CSP wt parasites at day 5 PI (Fig. 2f ). Interestingly, TEP1 was only observed to bind to the surface of CSP mut oocysts and co-localized with CSP protein inside the mutant oocysts, but not for CSP wt oocysts at day 7 PI (Fig. 2g ). When TEP1 was silenced, however, no oocysts were found to be melanized in CSP mut parasite-infected mosquitoes on day 12 PI (Fig. 2h ), and an increased number of CSP mut sporozoites appeared in the hemolymph (Fig. 2i ). Both the motility and infectivity of CSP mut hemolymph sporozoites were comparable to those of the CSP wt hemolymph sporozoites in vitro (Supplementary Movie 1 , 2 and Supplementary Fig. 2 ), indicating no biological defect in mutant parasites. The melanization of the killed parasites was initiated by melanin biosynthesis, which is mediated by PPO cascades [25] . In addition, only hemocyte-derived PPOs, such as PPO1, PPO2, PPO3, and PPO9, have been reported to mediate oocyst killing [15] , [26] . Therefore, we next investigated whether those PPOs were involved in this process. As a result, we found that TEP1 knockdown could only significantly downregulate the mRNA levels of PPO2 , PPO3 , and PPO9 , but not PPO1 , in mosquitoes infected with the CSP mut parasite (Supplementary Fig. 3 ), indicating the involvement of PPOs in the melanization of oocysts. Thus, the results demonstrated that the arrested development of CSP mut parasites was attributed to the TEP1-mediated killing of oocysts, which might involve PPOs. CSP mut infection induces hemocytes to release TEP1 in a Toll pathway-dependent manner We also found that more hemocytes were recruited to the midgut of mosquitoes infected with mutant parasites than those infected with WT parasites (Fig. 3a ). As cellular immune responses play an essential role in mosquito immunity [5] , the results further confirmed the ability of the mutant parasites to trigger mosquito immune defenses. Although a previous study argued that TEP1 was predominantly produced in the fat body [27] , more evidence has indicated hemocytes as the main source of TEP1 [26] , [28] . Therefore, we examined TEP1 expression in all three types of mosquito hemocytes: prohemocytes, granulocytes, and oenocytoids. No significant TEP1 expression was detected in prohemocytes from mosquitoes infected with either CSP mut or CSP wt parasites. However, as compared to CSP wt parasite-infected mosquitoes, a higher ratio of granulocytes from CSP mut parasite-infected mosquitoes expressed TEP1, as determined by either morphology identification (Fig. 3b ) or flow cytometry analysis of granulocytes (Supplementary Fig. 4 ). Chemical depletion of granulocytes using clodronate liposomes (CLDs) (Supplementary Fig. 5 ), as previously reported [26] , decreased both TEP1 expression and the percentage of melanized CSP mut oocysts but increased the number of hemolymph sporozoites (Fig. 3c ). Although flow cytometry could not accurately distinguish the TEP1-expressed oenocytoids from granulocytes (Supplementary Fig. 4 ), morphological identification suggested the upregulation of TEP1 in oenocytoids from CSP mut parasite-infected mosquitoes (Fig. 3b ). Thus, we demonstrated the essential role of hemocyte-derived TEP1 in the melanization of CSP mut oocysts. Fig. 3: Infection with CSP mut induces hemocytes to release TEP1 in a Toll-dependent manner. a The recruitment of hemocytes, which were stained with a hemocyte-specific lipophilic dye (Vybrant CM-DiI), to the midgut of mosquitoes at day 7 after infection with Plasmodium yoelii CSP wt or CSP mut parasites (left), and statistical analysis of hemocytes recruited to the midguts ( n = 64) (right); scale bar 50 μm. b A representative immunofluorescent confocal image of granulocyte, oenocytoid, and prohemocyte from P. yoelii CSP wt or CSP mut parasite-infected mosquitoes ( n = 60) at day 5 PI, stained with anti-TEP1 antibody (left), the percentage of TEP1 positive cells in granulocyte, oenocytoid, and prohemocyte was quantified (right). Scale bar 2 μm. c The percentage of melanized mature oocysts (left) in mosquitoes ( n = 45), the average number of hemolymph sporozoites (middle) in mosquitoes ( n = 45), and the expression of TEP1 (right) in mosquitoes ( n = 45) infected with P. yoelii CSP wt and CSP mut , pretreated with or without clodronate liposome. The mRNA levels of TEP1 in CSP mut parasite-infected mosquitoes ( n = 15) determined using real-time PCR, after GNBP-B1 ( d ) or Rel1 ( e ) knockdown. The percentage of melanized mature oocyst in CSP mut parasite-infected mosquitoes ( n = 45) determined after knockdown of GNBP-B1 ( f ) or Rel1 ( g ). The number of hemolymph sporozoites in CSP mut parasite-infected mosquitoes ( n = 45) counted after knockdown of GNBP-B1 ( h ) or Rel1 ( i ). For box-plot diagram ( a ): middle line represents median; boxes extend from the 25th to 75th percentiles. The whiskers mark the 10th and 90th percentiles. b , d – f A two-sided Student’s t -test was used for the statistical analysis. a , c , g – i A two-sided Mann–Whitney U test was used for the statistical analysis. The data were presented as the means ± SD; ns, no significance; p -values were shown. The data were combined based on three independent experiments ( a – i ). Source data are provided as a Source Data file. Full size image Next, we investigated the underlying mechanism of enhanced TEP1 expression in hemocytes induced by CSP mut parasite infection. 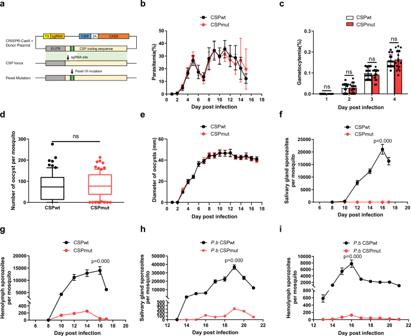Fig. 1: Release of sporozoites from CSPmutoocyst in mosquitoes is greatly impaired. aSchematic representing the construction of the recombinantPlasmodium yoeliiCSPmutparasite using CRISPR-Cas9. The amino acids of pexel I (RNLNE) and pexel II (RLLGD) in wild-type CSP were mutated into ANANA and ALAGA, respectively. Both the parasitemia (b) and gametocytemia (c) of mice (n= 15) infected with the CSPwtor CSPmutparasites were compared at the indicated time points. The average number of oocysts (d) in mosquitoes (n= 81) at day 7, and the average diameter of oocysts (e) under ×400 field in mosquitoes (n= 40) at the indicated time points after feeding on CSPwtor CSPmut-infected mice. The average number of salivary gland sporozoites (f) in mosquitoes (n= 90), and hemolymph sporozoites (g) in mosquitoes (n= 60) infected withP. yoeliiCSPwtor CSPmutparasites at the indicated time points were recorded. The average number of salivary gland sporozoites (h) in mosquitoes (n= 90), and hemolymph sporozoites (i) in mosquitoes (n= 60) infected withP. bergheiCSPwtor CSPmutparasites at the indicated time points. For box-plot diagram (d): middle line represents median; boxes extend from the 25th to 75th percentiles. The whiskers mark the 10th and 90th percentiles.c,dA two-sided Student’st-test was used for the statistical analysis.f–iA two-sided Mann–WhitneyUtest was used for the statistical analysis. The data were presented as the means ± SD; ns, no significance;p-values were shown. The data were combined based on three independent experiments (b–i). Source data are provided as a Source Data file. mRNA isolated from CSP wt and CSP mut parasite-infected mosquitoes at day 7 PI, 2 days before CSP mut oocyst melanization, was observed, sequenced, and compared (Supplementary Table 1 ). As TEP1 is reportedly regulated by the Toll, immune deficiency (IMD), and Janus kinase–STAT signaling pathways [23] , genes in each pathway were selected for comparison between CSP wt and CSP mut parasite-infected mosquitoes. No significant difference in the expression of IMD (ASTE010360), JNK (ASTE007551) and STAT (ASTE011642) involved in the IMD, JNK, and STAT signaling pathways was found between CSP wt - and CSP mut -infected mosquitoes. However, those belonging to the Toll signaling pathway, such as Gram-negative binding protein B1 ( GNBP-B1 ) (ASTE016199) and Relish-like protein 1 ( Rel1 ) (ASTE011378), were significantly upregulated (Supplementary Fig. 6a ), which was further validated by quantitative real-time PCR (Supplementary Fig. 6b ). Their roles in hemocyte TEP1 regulation during infection with CSP mut parasites were determined by RNA silencing. 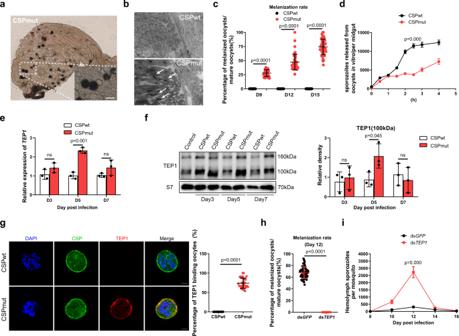Fig. 2: Parasite development arrest largely depends on TEP1-mediated mature CSPmutoocyst melanization. aRepresentative image of melanizedPlasmodium yoeliiCSPmutin mosquitoes under a light microscope on day 12 after a blood meal; scale bar 50 μm.bRepresentative electron micrograph of vacuolized or melanized sporozoites (white arrows) fromP. yoeliiCSPwtand CSPmutoocysts at day 11; scale bar 1 μm.cStatistical analysis between the percentage of melanized matureP. yoeliiCSPwtand CSPmutoocysts in mosquitoes (n= 45) at the indicated time points post blood feeding.dAverage number of sporozoites released fromP. yoeliiCSPwtand CSPmutoocysts in mosquitoes (n= 60) at indicated incubation times in vitro.emRNA expression level ofTEP1in mosquitoes (n= 15) infected withP. yoeliiCSPwtand CSPmutat the indicated time points post blood feeding determined using real-time PCR.fTEP1 activation (100 kD band) in hemocytes from mosquitoes (n= 40) infected withP. yoeliiCSPwtand CSPmutparasites detected using western blot; S7 protein was used as an internal control (left). Pooled data was quantified and analyzed (right).gRepresentative image of TEP1 binding toP. yoeliiCSPwtand CSPmutoocysts at day 7 PI stained with anti-CSP repeat and anti-TEP1 (left), and the percentage of oocysts fromP. yoeliiCSPwtor CSPmutparasite-infected mosquitoes (n= 30) bound with TEP1 was statistically analyzed (right); scale bar 10 μm. Percentage of melanized mature oocysts (h) inP. yoeliiCSPmutparasite-infected mosquitoes (n= 60) at day 12 PI, and average number of hemolymph sporozoites (i) in mosquitoes (n= 60) infected with CSPmutparasites at the indicated time points compared followingTEP1knockdown.d–fA two-sided Student’st-test was used for the statistical analysis.c,g–iA two-sided Mann–WhitneyUtest was used for the statistical analysis. The data were presented as the means ± SD; ns, no significance;p-values were shown. The data were combined based on three independent experiments (c–i) or two independent experiments (b). Source data are provided as a Source Data file. As a result, the inhibition of either JNK, STAT, or IMD signaling pathways by knockdown of the related genes, JNK (ASTE007551), STAT (ASTE011642), or IMD (ASTE010360), respectively, had no significant effect on the melanization of CSP mut oocysts (Supplementary Table 2 ). However, knockdown of Toll pathway-related genes, GNBP-B1 and Rel1 , significantly reduced TEP1 expression (Fig. 3d, e ), and inhibited CSP mut oocyst melanization (Fig. 3f, g ) but significantly increased the number of hemolymph sporozoites (Fig. 3h, i ). Thus, we demonstrated that infection with CSP mut parasites significantly induced TEP1 expression in a Toll pathway-dependent manner, which is closely associated with the melanization of mature mutant oocysts. CSP mut parasites trigger mosquito immune responses through the induction of hemocyte nitration Next, we investigated the underlying mechanism behind Toll pathway activation by CSP mut infection. Wolbachia infection in mosquitoes activates the Toll pathway by inducing the production of reactive oxygen species in Aedes aegypti ; [29] therefore, we selected antioxidant genes for analysis in mosquitoes infected with CSP wt or CSP mut parasites. Importantly, genes encoding heme peroxidase, such as HPX2 , DBLOX ( double heme peroxidase ), NOX5 , and DUOX ( dual oxidase ), were significantly upregulated in CSP mut -infected mosquitoes (Supplementary Fig. 7a, b ). HPX2 and NOX5 are critical for the nitration of ookinete-invaded midgut epithelial cells and trigger the mosquito immune response against parasites [1] . This prompted us to investigate whether infection with CSP mut parasites could induce the nitration of recruited hemocytes and elicit an immune response. A significantly higher level of nitration was observed in hemocytes around the oocysts of mosquitoes infected with CSP mut parasites, compared to the CSP wt parasite-infected mosquitoes (Fig. 4a ). Interestingly, some nitrated hemocytes were found to attach to the CSP mut oocysts (Supplementary Fig. 8 ) and simultaneously express TEP1 (Fig. 4a ), indicating that some hemocytes recruited to mutant oocysts might be activated to express TEP1. To investigate the molecular mechanism underlying hemocyte nitration induced by CSP mut parasite infection, we silenced the upregulated antioxidant genes ( NOX5 , DUOX , DBLOX , and HPX2 ) and determined the effect on hemocyte nitration. Knockdown of NOX5 abrogated the nitration of hemocytes in CSP mut -infected mosquitoes (Fig. 4a ) and resulted in the downregulation of GNBP-B1 , Rel1 , and TEP1 mRNA levels, and the disappearance of CSP mut oocyst melanization, increased the number of sporozoites in the hemolymph (Fig. 4b–d ), but the silencing of DUOX or DBLOX has no significant effect on the melanization of CSP mut oocysts (Supplementary Table 2 ). In contrast to the important role that HPX2 plays in the nitration of ookinete-invaded midgut epithelial cells, knockdown of HPX2 had no significant effect on hemocyte nitration, oocyst melanization, or the number of sporozoites in the hemolymph of CSP mut -infected mosquitoes (Supplementary Fig. 9 ). Therefore, infection with mutant parasites results in the nitration of hemocytes and elicits a mosquito immune response to limit parasite development. Fig. 4: CSP mut triggers mosquito immune responses through the induction of hemocyte nitration. a Representative image of the nitration and TEP1 expression of hemocytes around oocysts in Plasmodium yoelii CSP wt or CSP mut parasite-infected mosquitoes at day 4 after NOX5 was knocked down or not. This was determined by the detection of nitrotyrosine (NY), TEP1, and Vybrant CM-DiI (Dil); scale bar 50 μm (upper), and the numbers of nitrated hemocytes and TEP1-positive nitrated hemocytes attached to midguts ( n = 60) were statistically analyzed (low). Yellow arrow indicates either WT or mutant oocysts; white arrow indicates hemocytes. b The relative expression of TEP1 , GNBP-B1 , and Rel1 in P. yoelii CSP mut parasite-infected mosquitoes ( n = 15) at day 5 PI after NOX5 knockdown. c The percentage of melanized mature oocyst in P. yoelii CSP mut parasite-infected mosquitoes ( n = 36) at the indicated time points after NOX5 knockdown. d The average number of hemolymph sporozoites in P. yoelii CSP mut parasite-infected mosquitoes ( n = 45) at the indicated time points after NOX5 knockdown. For box-plot diagram ( a ): middle line represents median; boxes extend from the 25th to 75th percentiles. The whiskers mark the 10th and 90th percentiles. a , b A two-sided Student’s t -test was used for the statistical analysis. c , d A two-sided Mann–Whitney U test was used for the statistical analysis. The data were presented as the means ± SD; ns, no significance; p -values were shown. The data were combined based on three independent experiments ( a – d ). Source data are provided as a Source Data file. Full size image CSP conformation is altered in CSP mut parasites and induces hemocyte nitration It has been reported that CSP expression levels in oocysts affect sporozoite morphology [30] . This prompted us to investigate whether the developmental defect observed in CSP mut parasites was due to the reduced CSP expression. The expression of CSP could be detected as early as day 4 PI in midgut oocysts using real-time PCR and detected at day 5 PI using western blot (Supplementary Fig. 10 ). However, the expression levels of CSP in CSP wt oocysts was comparable to that observed in CSP mut oocysts (Fig. 5a and Supplementary Fig. 10 ). Thus, the effect of CSP expression on the developmental defects of CSP mut parasites could be excluded. Evidence has shown that CSP undergoes a conformational change when sporozoites are released from the oocyst into the hemolymph. The thrombospondin repeat domain (TSR) at the C-terminus of CSP is exposed at the surface of oocyst sporozoites but is masked at hemolymph sporozoites surface by the N-terminus [31] . We therefore speculated that the mutation of the pexel I/II domain at the CSP N-terminus may result in a conformational change. Although anti-C-terminal CSP polyclonal antibody detected oocysts and hemolymph sporozoites of both the WT and mutant parasites (Fig. 5b ), only mutant oocysts and hemolymph sporozoites were detected with anti-N-terminal CSP polyclonal antibody (Fig. 5b ). Thus, our results strongly suggest that the mutation of the pexel I/II domain resulted in a conformational change of the CSP N-terminus. We noted a slightly different pattern in the WT hemolymph sporozoites labelled by anti-C-terminal CSP polyclonal antibody between ours and a previous study [31] . This discrepancy may be explained by the smaller peptide of the C-terminus of CSP used for the preparation of the anti-sera in our experiment, whereas the full length TSR region in the C-terminus of CSP was used in the previous study [31] . Fig. 5: CSP conformation of CSP mut is altered and induces the nitration of hemocytes. a Representative image of CSP relative expression in Plasmodium yoelii CSP wt and CSP mut oocysts from mosquitoes ( n = 40) detected by western blot at days 7, 9, and 12 post blood meal (upper); CSP relative expression was statistically analyzed (lower). b Representative immunofluorescence image of oocyst (scale bar 10 μm) and hemolymph sporozoites (scale bar 5 μm) from P. yoelii CSP wt or CSP mut parasite-infected mosquitoes stained with anti-CSP-N and anti-CSP-C terminal antibodies. c Representative immunofluorescence image of in vitro nitration of hemocytes from naïve mosquitoes ( n = 20) stimulated by midguts ( n = 20) from P. yoelii CSP wt or CSP mut parasite-infected mosquitoes at day 5 PI (left). WGA was used to distinguish hemocytes, and hemocyte nitration was determined using anti-nitrotyrosine staining; scale bar 5 μm. Percentage of the nitrated hemocytes was statistically analyzed (right). d GNBP-B1 , Rel1 , and TEP1 expression in hemocytes from naïve mosquitoes ( n = 20) following incubation with midguts ( n = 20) from P. yoelii CSP wt or CSP mut parasite-infected mosquitoes at day 5 PI determined using real-time PCR. e Representative immunofluorescence image of the nitration of hemocytes from naïve mosquitoes ( n = 20) incubated with midguts from P. yoelii CSP mut parasite-infected mosquitoes ( n = 20) at day 5 PI with or without NOX5 silenced (left); scale bar 5 μm. Hemocyte nitration was determined as described in c and statistically analyzed (right). f GNBP-B1 , Rel1 , and TEP1 expression in hemocytes from naïve mosquitoes ( n = 20) with or without ds NOX5 incubated with midguts ( n = 20) from P. yoelii CSP mut parasite-infected mosquitoes at day 5 PI. A two-sided Student’s t -test was used for the statistical analysis. The data were presented as the means ± SD; ns, no significance; p -values were shown. The data were combined based on three independent experiments ( a , c – f ) or two independent experiments ( b ). Source data are provided as a Source Data file. Full size image To test whether this CSP conformational change triggers the nitration of hemocytes recruited to midgut basal lamina, both WT and mutant oocysts were incubated with hemocytes from naïve mosquitoes, and hemocyte nitration was determined. A higher number of hemocytes were found to be nitrated when incubated with mutant oocysts than with CSP wt oocysts (Fig. 5c ). Furthermore, much higher expression levels of GNBP-B1 , Rel1 , and TEP1 were detected in hemocytes stimulated with CSP mut oocysts (Fig. 5d ). However, nitration and enhanced expression of GNBP-B1 , Rel1 , and TEP1 were abrogated in NOX5-silenced hemocytes when incubated with CSP mut oocysts (Fig. 5e, f ). Thus, our findings demonstrated that the NOX5-mediated nitration of hemocytes and the mosquito immune response were elicited by the CSP conformational change in CSP mut parasites. Pre-infection of mosquitoes with CSP mut reduces parasite burden when challenged with RFP-expressing WT parasites To further confirm that the mosquito immune response can be elicited by these mutant parasites, mosquitoes were first infected with CSP wt or CSP mut and then challenged with a red fluorescent protein (RFP)-expressing WT parasite (265BY P. yoelii -RFP) at day 3 PI. This time point was selected for the re-challenge because a robust mosquito immune response was stimulated by mutant oocyst CSP and mainly targeted oocysts of the re-challenged parasite. After the RFP-expressing WT parasite re-challenged at day 3 PI developed into early oocysts, the firstly infected mutant parasites were developed for approximately 5 days. At that time, the developed mutant oocysts would trigger mosquito immune responses against the re-challenged parasites. Although the number of 265BY P. yoelii -RFP oocysts was comparable between mosquitoes pre-infected with CSP mut and CSP wt parasites (Fig. 6a ), oocyst melanization in pre-infected mosquitoes began at day 9 PI, and the percentage of melanized oocysts increased from 16% on day 9 to 67%, on day 15 PI (Fig. 6b ). Here, it should be noted that the definitive origin of melanized oocysts was difficult to determine, as the fluorescence could be faded as the RFP-expressing oocyst was melanized. We observed the melanized RFP-expressing oocyst at both light and fluorescent microscopy and found some melanized oocyst could still be identified by residual fluorescence (Fig. 6b ). However, some melanized RFP-expressing oocysts without residual fluorescence could have been missed. Therefore, the actual percentage of the melanized RFP-expressing oocysts should be higher than what we have reported here. As a result, fewer RFP-expressing hemolymph and salivary gland sporozoites were observed in mosquitoes pre-infected with CSP mut , as compared to those pre-infected with the CSP wt parasites (Fig. 6c, d ). This indicates that mosquitoes pre-infected with CSP mut parasites develop resistance to re-challenge with the RFP-expressing WT parasite. Fig. 6: Pre-infection of mosquitoes with CSP mut reduces parasite burden when challenged with RFP-expressing WT parasites. Mosquitoes infected with Plasmodium yoelii CSP wt or CSP mut parasites were re-challenged with P. yoelii -RFP 3 days after the first blood meal. a The average number of P. yoelii -RFP oocysts in mosquitoes ( n = 60) pre-infected with or without P. yoelii CSP wt or CSP mut parasite at day 7 PI. b A representative image of P. yoelii oocysts in mosquitoes pre-infected with P. yoelii CSP wt or CSP mut parasites under the light microscope and using immunofluorescence, respectively (left); the percentage of melanized oocysts in mosquitoes ( n = 36) pre-infected with P. yoelii CSP wt or CSP mut parasites at the indicated time points were compared (right); scale bar 50 μm. The average number of hemolymph sporozoites ( c ) in mosquitoes ( n = 45), and salivary gland sporozoites ( d ) in mosquitoes ( n = 90) pre-infected with P. yoelii CSP wt or CSP mut parasites were compared at the indicated times. The average number of P. yoelii -RFP oocysts ( e ) in mosquitoes ( n = 60), the percentage of melanized oocysts ( f ) in mosquitoes ( n = 36), the average number of hemolymph sporozoites ( g ) in mosquitoes ( n = 45), and salivary gland sporozoites ( h ) in mosquitoes ( n = 60) pre-infected with CSP mut parasite were compared after NOX5 knockdown. i The mRNA levels of TEP1 , GNBP-B1 , and Rel1 in mosquitoes ( n = 15) pre-infected with P. yoelii CSP mut parasites at day 5 PI after NOX5 knockdown were determined using real-time PCR. For box-plot diagram ( a , e ): middle line represents median; boxes extend from the 25th to 75th percentiles. The whiskers mark the 10th and 90th percentiles. A two-sided Student’s t -test was used for the statistical analysis. The data are presented as the means ± SD; ns, no significance; p -values are shown. The data were combined based on three independent experiments ( a – i ). Source data are provided as a Source Data file. Full size image To test whether hemocyte nitration contributed to the resistance observed in CSP mut pre-infected mosquitoes, NOX5 was silenced prior to infection with 265BY P. yoelii -RFP. Following NOX5 knockdown, melanization of RFP-expressing WT oocysts disappeared, although no change in oocyst number was observed (Fig. 6e, f ). In addition, the number of hemolymph sporozoites increased, and a few infectious salivary gland sporozoites appeared (Fig. 6g, h ). In addition, NOX5 knockdown significantly inhibited TEP1 expression and downregulated the genes of the Toll pathway (Fig. 6i ). Therefore, we demonstrated that CSP mut infection triggered the mosquito immune defense by inducing nitration, and CSP might be explored as a potential target to block malaria transmission. Compared to the great loss of parasites that occurs during ookinete penetration of the mosquito midgut epithelium, only a small proportion of parasites are lost during the oocyst stage [32] . This indicates that oocysts tend to evade mosquito immune defenses; however, the underlying mechanism is still unknown. In the present study, we demonstrated that CSP, on the inner membrane of oocysts and the surface of sporozoites [30] , is required for the evasion of mosquito immune responses. The change in CSP conformation through mutation of the pexel I/II domain made the parasite visible to the mosquito immune system through the induction of hemocyte nitration. Although previous studies have shown that the mosquito immune response can limit oocyst development [12] , [13] , [14] , [15] , [33] , oocysts are less vulnerable than ookinetes to the mosquito immune system [16] . This indicates that oocysts have evolved strategies to escape mosquito immunity to facilitate their survival. The incorporation of mosquito proteins such as laminin, matrix metalloprotease 1 (MMP1), and lysozyme c-1 (LYSC-1) into the oocyst capsule might represent an effort by the oocyst to mask itself with mosquito self-proteins to evade immune recognition [34] , [35] . A similar strategy is used by gametes that cover their surface with human factor H, which is present in the blood bolus, to evade human complement in the mosquito midgut [36] . In the present study, we found that oocysts could use their own protein, CSP, to avoid mosquito immune recognition. Previously, Pfs47 on the ookinetes of mosquito-susceptible P. falciparum strain was demonstrated to block the JNK pathway to foster parasite development in the mosquito [11] . In contrast to Pfs47 , concealing CSP is a strategy used by malaria parasite oocysts to evade host immunity as the mutation of the CSP pexel I/II domain of either P. yoelii or P. berghei resulted in the developmental arrest of mature oocysts (Fig. 1 ). We found that the CSP pexel I/II domain mutation resulted in a conformational change (Fig. 5 ), which induced nitration of hemocytes attached to the midgut, and triggered mosquito immune responses. A similar phenomenon was observed when midgut epithelial cells were invaded by ookinetes, and it could be elicited by the exposure of epithelium intracellular molecules, which were sensed as danger signal by mosquito immunity [4] . Although the definitive mechanism by which the mutant parasite induces hemocyte nitration remains unknown, we postulated that the conformational change in CSP might change the physical surface of oocysts, which would be sensed by the circulating hemocytes because nitrated hemocytes were found to attach to mutant oocysts (Supplementary Fig. 8 ). After the hemocytes were activated, TEP1 released by hemocytes could more easily permeate into the mutant oocyst, as supported by our observation of the co-localization of TEP1 with CSP inside the oocyst (Fig. 2g ). Although both NOX5 and HPX2 are essential for the nitration of ookinete-invaded midgut epithelium, only NOX5 was involved in the nitration reaction induced by mutant parasites (Fig. 4 and Supplementary Fig. 9 ), indicating that some differences might exist between these two mechanisms. Previous research has demonstrated that CSP is required for sporozoite formation in oocysts through the disruption of the CS gene [37] . Another study showed that the lack of a repeated region, with or without the N-terminus, resulted in a defect in sporozoite development [38] . However, the deletion of the N-terminus (ΔNfull CSP mutant), or mutation of region II plus in the C-terminus of CSP, did not affect sporozoite formation in oocysts but severely reduced the release of sporozoites from mutant oocysts [31] , [39] . In contrast, we revealed that CSP plays a role in the modulation of mosquito immune responses when its pexel I/II domain was mutated, which has not been reported in previous studies [31] , [38] , [39] . This discrepancy might be explained by the fact that different CSP domains were mutated in our study, and that CSP immune evasion may have been masked when the N-terminus or repeated region was deleted, or region II plus in the C-terminus was mutated in previous studies [31] , [38] , [39] . Alternatively, the melanization of mutant parasites might have been missed in previous studies [31] , [38] , [39] . Therefore, we described a dual function for CSP, including immune evasion and sporogonic development. Our finding is supported by a recently identified ookinete and sporozoite surface protein, Plasmodium Infection of the Mosquito Midgut Screen 43 (PIMMS43), which is also required for parasite evasion of the mosquito complement-like response, as well as sporogonic development in the oocyst [40] . We also noted that the number of sporozoites in the hemolymph from CSP mut parasite oocysts did not return to CSP wt parasite levels, even when the melanization of mutant oocysts was completely abrogated. As CSP plays a critical biological role in parasite development in mosquitoes, the effects of CSP pexel I/II domain mutation on sporozoite release from oocysts could not be completely excluded. Further, in addition to the conformational change in CSP in the inner membrane of the oocyst, the conformation of CSP on hemolymph sporozoites also varied (Fig. 5 ), which might induce a more robust mosquito immune response than that of CSP wt sporozoites. As a result, more mutant sporozoites might be cleared from the hemolymph than CSP wt sporozoites. However, this needs to be confirmed in future studies. In conclusion, we found that mutation of the CSP pexel I/II domain induced the nitration of hemocytes, which subsequently recruited additional hemocytes to the midgut basal lamina. Furthermore, nitration enhanced the expression of TEP1 in hemocytes in a Toll-dependent manner, induced melanization of mature oocysts, and resulted in the impaired release of sporozoites from the CSP mut oocysts (Fig. 7 ). Thus, we described a TEP1-dependent immune response elicited by the recognition of mutant mature oocysts. In contrast, previous studies have reported a significant loss in parasite numbers between the early and mature oocyst stages mediated by mosquito hemocytes [8] , [14] , [15] and PPOs [14] , [15] but independent of TEP1 function [13] , [41] . Therefore, our findings might represent an additional mechanism by which oocysts can be recognized and targeted in the mosquito. However, it is possible that the differences in the immune response between ours and previous studies were due to the different strains of Anopheles used. CSP is regarded as the predominant protective antigen of the irradiation-attenuated sporozoites [42] , and the main component of the leading liver-stage subunit vaccine RTS,S [43] , [44] . Our results highlight CSP also as a potential target for malaria transmission-blocking vaccines. Fig. 7: Schematic illustration showing how CSP mut parasites trigger mosquito immune responses. CSP mut oocysts, with a conformational change in the inner membrane protein CSP due to a mutation in its pexel I/II domain, induce the nitration of hemocytes attached to the midgut and enhance the expression of TEP1 in a Toll pathway-dependent manner. The binding of TEP1 to oocysts results in the melanization or vacuolation of mature oocysts, and the release of sporozoites from the CSP mut oocysts was impaired. Full size image Malaria parasites, mosquitoes and mice Both P. yoelii 265BY and P. yoelii 265BY-RFP, which was constructed using a single cross-mediated insertion of RFP in the SSU rRNA gene of the P. yoelii 265BY parasite [45] , were maintained by alternate passaging between Kunming mice (Army Medical University, Chongqing, China) and Anopheles stephensi in our laboratory. P. berghei ANKA was donated by Dr. Xin-Zhuan Su (NIAID, MD, USA). A. stephensi from our laboratory was maintained at 27 °C at a relative humidity of 70–80%, and fed with a 10% sugar solution containing 0.5% para-aminobenzoic acid (PABA). The room was on a cycle of 12 h light/dark (lights off at 18:00).Kunming mice (Female, 6–8 weeks old) were provided by the Laboratory Animal Center of the Army medical University (Chongqing, China); BALB/c and C57BL/6 J mice (Female, 6–8 weeks old) purchased from Beijing Animal Institute (Beijing, China). The mice were kept in a temperature- and humidity-controlled room on a cycle of 12 h light/dark (lights off at 19:00). All animal protocols were reviewed and approved by the Animal Ethics Committee of the Army Medical University Institute of Medical Research (AMUWEC20181777). Construction of the CSP mutant parasites Using CRISPR-Cas9 technology, P. yoelii 265BY parasites were generated by replacing the P. yoelii 265BY WT CSP sequence with a mutated CSP pexel I/II domain sequence (the sequences of pexel I and pexel II were mutated into ANANA and ALAGA, respectively), as previously reported [18] . Briefly, a single guide RNA (5'-GATTCTCTACTTCCAGGATA-3') specifically targeting the P. yoelii 265BY CSP gene (GenBank Gene ID: DQ012939.1) was inserted downstream of the Plasmodium U6 promoter in the pYC plasmid (donated by Dr. Jing Yuan, Xia’men University, China). The homologous recombinant fragment, containing a 5' untranslated region (551 bp) and a fragment encoding the mutated CSP pexel I/II domain (1284 bp), was constructed by overlapping PCR and then inserted into the multiple cloning sites of the pYC plasmid (Supplementary Fig. 1 ). The resulting pYC-CSP mut recombinant plasmid was amplified, purified using the E.Z.N.A ® Endo-Free Plasmid Midi Kit (Omega Bio-Tek, GA, USA), and electroporated into synchronic schizont cultures as previously reported [46] . Following electroporation, the transfection medium was immediately injected into the tail vein of Kunming mice. Once parasites appeared in the blood, mice were fed pyrimethamine (6 μg/mL; Sigma-Aldrich, St. Louis, MO, USA). The pyrimethamine-resistant parasites were harvested, and then each mouse was injected intravenously with 100 μL of parasite solution diluted with ~1.0 infected red blood cell in phosphate-buffered saline (PBS) to clone pyrimethamine-resistant parasites. After 7–9 days, blood from mice with cloned parasites was harvested, and genomic DNA was extracted. The mutated CSP mut was identified using PCR and then verified using DNA sequencing (Supplementary Fig. 1 ). The construction of the CSP mutant in P. berghei ANKA parasites was performed as previously described [19] . Infection of mice with malaria parasites Female 6–8-week-old BALB/c mice (5 mice each group) were intravenously infected with 1 × 10 6 P. yoelii 265BY CSP wt or CSP mut parasitized red blood cells (pRBCs) and P. berghei ANKA CSP wt or CSP mut pRBCs, and the parasitemia and gametocytemia were recorded daily. Mosquito infection For infection with CSP wt or CSP mut , 3–5-day-old female A. stephensi mosquitoes were allowed to feed on BALB/c mice (3–5 mice each group) displaying over 0.1% gametocytemia, and then fed with a 10 % sugar solution at 23–24 °C. On day 7, mosquito midguts were dissected to determine the oocyst burden. Hemolymph was harvested on days 8–15 to determine the number of hemolymph sporozoites, and salivary glands were dissected at day 17 post blood meal. Quantitative real-time PCR analysis Total RNA was extracted from either CSP wt - or CSP mut -infected mosquitoes using TRIzol TM Reagent (Thermo Fisher Scientific, Waltham, MA, USA) following the manufacturer’s instructions. The quality and concentration of each RNA sample were determined using a NanoDrop One Spectrophotometer (Thermo Fisher Scientific), and 2 µg RNA was used for first-strand cDNA synthesis with the PrimeScript™ RT reagent Kit with gDNA Eraser (Perfect Real Time) (Takara Bio Inc., Japan). 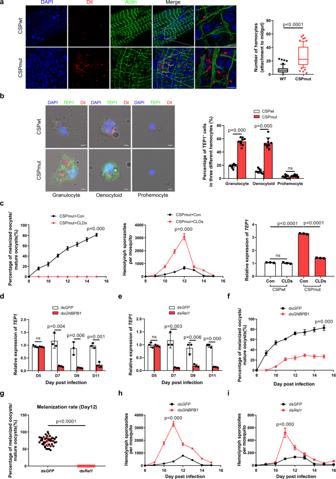Fig. 3: Infection with CSPmutinduces hemocytes to release TEP1 in a Toll-dependent manner. aThe recruitment of hemocytes, which were stained with a hemocyte-specific lipophilic dye (Vybrant CM-DiI), to the midgut of mosquitoes at day 7 after infection withPlasmodium yoeliiCSPwtor CSPmutparasites (left), and statistical analysis of hemocytes recruited to the midguts (n= 64) (right); scale bar 50 μm.bA representative immunofluorescent confocal image of granulocyte, oenocytoid, and prohemocyte fromP. yoeliiCSPwtor CSPmutparasite-infected mosquitoes (n= 60) at day 5 PI, stained with anti-TEP1 antibody (left), the percentage of TEP1 positive cells in granulocyte, oenocytoid, and prohemocyte was quantified (right). Scale bar 2 μm.cThe percentage of melanized mature oocysts (left) in mosquitoes (n= 45), the average number of hemolymph sporozoites (middle) in mosquitoes (n= 45), and the expression of TEP1 (right) in mosquitoes (n= 45) infected withP. yoeliiCSPwtand CSPmut, pretreated with or without clodronate liposome. The mRNA levels ofTEP1in CSPmutparasite-infected mosquitoes (n= 15) determined using real-time PCR, afterGNBP-B1(d) orRel1(e) knockdown. The percentage of melanized mature oocyst in CSPmutparasite-infected mosquitoes (n= 45) determined after knockdown ofGNBP-B1(f) orRel1(g). The number of hemolymph sporozoites in CSPmutparasite-infected mosquitoes (n= 45) counted after knockdown ofGNBP-B1(h) orRel1(i). For box-plot diagram (a): middle line represents median; boxes extend from the 25th to 75th percentiles. The whiskers mark the 10th and 90th percentiles.b,d–fA two-sided Student’st-test was used for the statistical analysis.a,c,g–iA two-sided Mann–WhitneyUtest was used for the statistical analysis. The data were presented as the means ± SD; ns, no significance;p-values were shown. The data were combined based on three independent experiments (a–i). Source data are provided as a Source Data file. The resulting cDNA was then used as a template for subsequent quantitative real-time PCR (qPCR) using the TB Green ® Premix Ex Taq™II (Tli RNaseH Plus) (Takara Bio Inc.) with target-specific primers (Supplementary Table 3 ). The assay was run on a CFX96 Real-Time PCR Detection System (Bio-Rad, Hercules, CA, USA), and relative quantitative results were normalized to the ribosomal protein S7 gene which was used as an internal control. dsRNA synthesis and gene silencing All the dsRNA products for silencing genes such as TEP1 , Rel1 , GNBP-B1 , and NOX5 were generated using a cDNA template from A. stephensi , and the MEGAscript TM RNAi Kit (Thermo Fisher Scientific) as previously described [3] , [7] . In brief, 3-day-old female A. stephensi were cold-anesthetized and injected with 3 mg/mL of dsRNA using a Nanoject II injector (Drummond Scientific Co., Broomall, PA, USA), 2 days prior to infection. Silencing efficiency was examined at day 2 post-knockdown by qPCR, as described above. Primers designed for specific transcript targets are listed in Supplementary Table 3 . Electron microscopy Midguts dissected from infected mosquitoes at day 11 after blood meal were fixed with 2.5% (v/v) glutaraldehyde in 0.05 M PBS (pH 7.4) with 4% sucrose for 12 h, and post-fixed in 1% osmium tetroxide for 1 h. After 30 min of en bloc staining with 1% aqueous uranyl acetate, the midgut tissues were dehydrated in ascending concentrations of ethanol and embedded in Epon 812. Ultrathin sections were stained with 2% uranyl acetate in 50% methanol and lead citrate and then observed under an electron microscope (Zeiss CEM 902; Zeiss Group, Oberkochen, Germany). Polyclonal antibody preparation Anti-CSP-N, anti-CSP-C, anti-CSP-repeat-region, and anti-TEP1 were synthesized by GeneCreate Biotech (Wuhan, China). 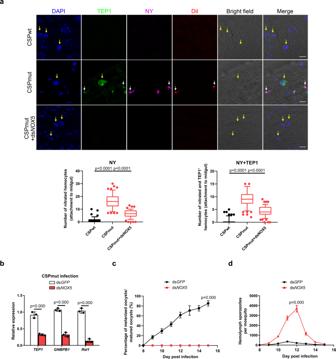Fig. 4: CSPmuttriggers mosquito immune responses through the induction of hemocyte nitration. aRepresentative image of the nitration and TEP1 expression of hemocytes around oocysts inPlasmodium yoeliiCSPwtor CSPmutparasite-infected mosquitoes at day 4 afterNOX5was knocked down or not. This was determined by the detection of nitrotyrosine (NY), TEP1, and Vybrant CM-DiI (Dil); scale bar 50 μm (upper), and the numbers of nitrated hemocytes and TEP1-positive nitrated hemocytes attached to midguts (n= 60) were statistically analyzed (low). Yellow arrow indicates either WT or mutant oocysts; white arrow indicates hemocytes.bThe relative expression ofTEP1,GNBP-B1, andRel1inP. yoeliiCSPmutparasite-infected mosquitoes (n= 15) at day 5 PI afterNOX5knockdown.cThe percentage of melanized mature oocyst inP. yoeliiCSPmutparasite-infected mosquitoes (n= 36) at the indicated time points afterNOX5knockdown.dThe average number of hemolymph sporozoites inP. yoeliiCSPmutparasite-infected mosquitoes (n= 45) at the indicated time points afterNOX5knockdown. For box-plot diagram (a): middle line represents median; boxes extend from the 25th to 75th percentiles. The whiskers mark the 10th and 90th percentiles.a,bA two-sided Student’st-test was used for the statistical analysis.c,dA two-sided Mann–WhitneyUtest was used for the statistical analysis. The data were presented as the means ± SD; ns, no significance;p-values were shown. The data were combined based on three independent experiments (a–d). Source data are provided as a Source Data file. Polypeptide and antigenic sequences designed for specific antibodies are listed in Supplementary Table 4 . Peptides were purified by high-performance liquid chromatography (HPLC) on a Waters Corporation Prominence HPLC system (Milford, MA, USA), using a Waters X Bridge C18 column (4.6 × 250 mm × 5 µm; Waters Corporation), and then conjugated to bovine serum albumin (BSA). The conjugated peptides were emulsified with Freund’s adjuvant (Sigma-Aldrich) and used to immunize specific-pathogen-free rabbits at 0, 2, 4, and 6 weeks. Seven days after the last immunization, serum was collected, and the antibody titers were determined using enzyme-linked immunosorbent assay (cat. no. 44-2404-21, Nunc 584 MaxiSorp flat bottom, Nalge Nunc International, Penfield, NY, USA). Protein G Sepharose (GE Healthcare, Chicago, IL, USA) was used to purify the polyclonal antibodies. For anti- P. yoelii HSP70 and anti-mosquito S7 polyclonal antibody preparation, the coding sequences of P. yoelii HSP70 (GenBank No. PY17X_0712100) and A. stephensi S7 (VectorBase Gene ID: ASTE004816) were separately cloned into pCzn1 (Zoonbio, Nanjing, China), and pET B2M (GeneCreate Biotech, Wuhan, China) expression vector, and the expression of both HSP70 and S7 in E. coli Arctic-ExpressTM was induced by IPTG, and the protein was purified by Ni column. New Zealand white rabbits were immunized with Hsp70 protein or S7 protein as antigen. After 3-4 rounds of immunization, the specific polyclonal antibody against HSP70 or S7 was purified by antigen affinity purification column, and the titer, purity, and concentration of the purified antibody were detected by ELISA. Experiments were carried out by Zoonbio and GeneCreate Biotech. Immunofluorescence analysis Hemocytes were harvested from mosquitoes infected with either CSP wt or CSP mut on day 5 post blood meal and used for the detection of TEP1 expression. To detect the change in CSP conformation, oocysts and hemolymph sporozoites were collected from mosquitoes infected with CSP wt or CSP mut on days 7 and 12 post blood meal, respectively. The hemocytes and sporozoites were then mounted on glass slides treated with poly-L-lysine and fixed with 4% paraformaldehyde for 1 h. The midguts for oocyst staining were directly transferred into EP tubes for fixation. All samples were washed, blocked with PBS/BSA, and incubated with primary antibodies diluted (1:200) in PBS at 4 °C overnight. Samples were washed 2–3 times with PBS and incubated for 2 h at room temperature with Cy3-labeled or Alexa 488-conjugated secondary antibodies (Beyotime Biotech, Nantong, China) diluted (1:500) in PBS. The following primary antibodies were used: anti-CSP-N, anti-CSP-C, anti-CSP-repeat region, and anti-TEP1. Cell nuclei were counterstained with 4,6-diamidino-2-Phenylindole (DAPI; Beyotime Biotech). 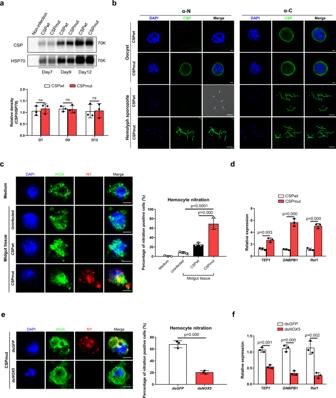Fig. 5: CSP conformation of CSPmutis altered and induces the nitration of hemocytes. aRepresentative image of CSP relative expression inPlasmodium yoeliiCSPwtand CSPmutoocysts from mosquitoes (n= 40) detected by western blot at days 7, 9, and 12 post blood meal (upper); CSP relative expression was statistically analyzed (lower).bRepresentative immunofluorescence image of oocyst (scale bar 10 μm) and hemolymph sporozoites (scale bar 5 μm) fromP. yoeliiCSPwtor CSPmutparasite-infected mosquitoes stained with anti-CSP-N and anti-CSP-C terminal antibodies.cRepresentative immunofluorescence image of in vitro nitration of hemocytes from naïve mosquitoes (n= 20) stimulated by midguts (n= 20) fromP. yoeliiCSPwtor CSPmutparasite-infected mosquitoes at day 5 PI (left). WGA was used to distinguish hemocytes, and hemocyte nitration was determined using anti-nitrotyrosine staining; scale bar 5 μm. Percentage of the nitrated hemocytes was statistically analyzed (right).dGNBP-B1,Rel1, andTEP1expression in hemocytes from naïve mosquitoes (n= 20) following incubation with midguts (n= 20) fromP. yoeliiCSPwtor CSPmutparasite-infected mosquitoes at day 5 PI determined using real-time PCR.eRepresentative immunofluorescence image of the nitration of hemocytes from naïve mosquitoes (n= 20) incubated with midguts fromP. yoeliiCSPmutparasite-infected mosquitoes (n= 20) at day 5 PI with or withoutNOX5silenced (left); scale bar 5 μm. Hemocyte nitration was determined as described incand statistically analyzed (right).fGNBP-B1,Rel1, andTEP1expression in hemocytes from naïve mosquitoes (n= 20) with or without dsNOX5incubated with midguts (n= 20) fromP. yoeliiCSPmutparasite-infected mosquitoes at day 5 PI. A two-sided Student’st-test was used for the statistical analysis. The data were presented as the means ± SD; ns, no significance;p-values were shown. The data were combined based on three independent experiments (a,c–f) or two independent experiments (b). Source data are provided as a Source Data file. Microscope slides were mounted using Dako Fluorescence Mounting Medium (Agilent). Observation of hemocytes attached to the midgut basal lamina To investigate the recruitment of hemocytes to the basal laminal of the midgut of mosquitoes infected with the CSP mut , 3–5-day-old A. stephensi were injected with 69 nL of 100 µM Vybrant ® CM-DiI cell labeling solution (Thermo Fisher Scientific), the day prior to gene-silencing experiments, as previously described [5] . To maintain the attachment of hemocytes to the midgut, 276 nL of 16% paraformaldehyde was injected into the anesthetized mosquitoes. The mosquitoes were allowed to stand for 40 s, and then the midgut was dissected in a 4% paraformaldehyde solution, and further fixed with 4% paraformaldehyde overnight at 4 °C. The following day, the midguts were washed twice with PBS, blocked with PBS containing 1% BSA for 40 min, and washed twice with the same solution. For actin and nuclei staining, midguts were incubated for 30 min at room temperature with 1 U of Alexa Fluor ® 647 phalloidin (Thermo Fisher Scientific), and DAPI (Beyotime Biotech). Tissues were mounted on microscope slides using Dako Fluorescence Mounting Medium (Agilent). 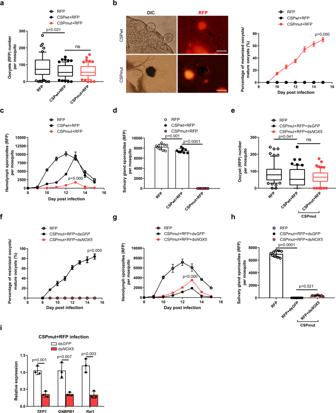Fig. 6: Pre-infection of mosquitoes with CSPmutreduces parasite burden when challenged with RFP-expressing WT parasites. Mosquitoes infected withPlasmodium yoeliiCSPwtor CSPmutparasites were re-challenged withP. yoelii-RFP 3 days after the first blood meal.aThe average number ofP. yoelii-RFP oocysts in mosquitoes (n= 60) pre-infected with or withoutP. yoeliiCSPwtor CSPmutparasite at day 7 PI.bA representative image ofP. yoeliioocysts in mosquitoes pre-infected withP. yoeliiCSPwtor CSPmutparasites under the light microscope and using immunofluorescence, respectively (left); the percentage of melanized oocysts in mosquitoes (n= 36) pre-infected withP. yoeliiCSPwtor CSPmutparasites at the indicated time points were compared (right); scale bar 50 μm. The average number of hemolymph sporozoites (c) in mosquitoes (n= 45), and salivary gland sporozoites (d) in mosquitoes (n= 90) pre-infected withP. yoeliiCSPwtor CSPmutparasites were compared at the indicated times. The average number ofP. yoelii-RFP oocysts (e) in mosquitoes (n= 60), the percentage of melanized oocysts (f) in mosquitoes (n= 36), the average number of hemolymph sporozoites (g) in mosquitoes (n= 45), and salivary gland sporozoites (h) in mosquitoes (n= 60) pre-infected with CSPmutparasite were compared afterNOX5knockdown.iThe mRNA levels ofTEP1,GNBP-B1, andRel1in mosquitoes (n= 15) pre-infected withP. yoeliiCSPmutparasites at day 5 PI afterNOX5knockdown were determined using real-time PCR. For box-plot diagram (a,e): middle line represents median; boxes extend from the 25th to 75th percentiles. The whiskers mark the 10th and 90th percentiles. A two-sided Student’st-test was used for the statistical analysis. The data are presented as the means ± SD; ns, no significance;p-values are shown. The data were combined based on three independent experiments (a–i). Source data are provided as a Source Data file. 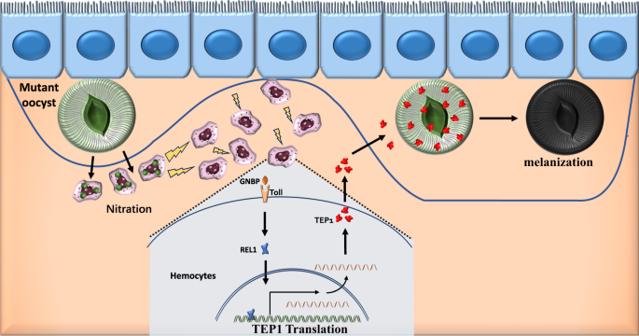Fig. 7: Schematic illustration showing how CSPmutparasites trigger mosquito immune responses. CSPmutoocysts, with a conformational change in the inner membrane protein CSP due to a mutation in its pexel I/II domain, induce the nitration of hemocytes attached to the midgut and enhance the expression of TEP1 in a Toll pathway-dependent manner. The binding of TEP1 to oocysts results in the melanization or vacuolation of mature oocysts, and the release of sporozoites from the CSPmutoocysts was impaired. Hemocytes were visualized by confocal microscopy (Leica TCS SP8) and LAS AF Lite was used for image acquisition and export, the number of hemocytes per midgut in each biological condition was analyzed. Nitration assay For immunofluorescence analysis of nitration in hemocytes attached to the midgut basal lamina, Vybrant ® CM-DiI cell labeling solution were injected into mosquitoes, and the midgut was dissected and fixed as described above. The following day, midguts were washed twice with PBS, blocked with PBS containing 1% BSA for 40 min, and washed twice with the same solution. The midguts were incubated overnight at 4 °C with diluted mouse anti-nitrotyrosine primary antibody (Abcam, Burlingame, CA, USA) diluted in PBS (1:500). Samples were then washed 2–3 times with PBS and incubated for 1 h at room temperature with Alexa 647-conjugated secondary antibodies (Beyotime Biotech) diluted (1:200) in PBS. Then, midguts were incubated with anti-TEP1 antibody diluted in PBS (1:200) for 3 h at room temperature. Samples were then washed 2–3 times with PBS and incubated for 1 h at room temperature with Alexa 488-conjugated secondary antibodies (Beyotime Biotech) diluted (1:500) in PBS. For nuclei staining, midguts were incubated for 5 min at room temperature with DAPI (Beyotime Biotech). Tissues were mounted on microscope slides using Dako Fluorescence Mounting Medium (Dako). In vitro assay of oocyst sporozoite release Midguts were dissected from either CSP wt - or CSP mut -infected mosquitoes on day 9 post blood meal. For each experiment, 20 midguts were incubated at 23 °C in 200 μL of RPMI medium. The solution (10 μL) was removed every 30 min, and the sporozoites released in the supernatant were quantified with a hemocytometer. Western blot analysis For the detection of TEP1 activation, hemolymph was collected from mosquitoes ( n = 20) infected with CSP wt or CSP mut on days 3, 5, and 7 after blood meal. For the detection of CSP expression, oocysts from CSP wt or CSP mut parasite-infected mosquito midguts ( n = 40) were collected on days 4, 5, 7, 9, and 12 post blood meal. Samples were dissolved in T-PER Tissue Protein Extraction Reagent (Thermo Fisher Scientific) containing a Halt Protease & Phosphatase Inhibitor Cocktail (Thermo Fisher Scientific). Protein samples (~20 µg) were mixed with Laemmli Sample Buffer (Bio-Rad), heated at 100 °C for 10 min, and then separated on a 10% TGX Stain-Free FastCast TM Acrylamide Kit (Bio-Rad). The separated proteins were transferred to a PVDF membrane and blocked in BSA for 1 h at room temperature. For the detection of TEP1 activation, the membrane was then incubated with a 1:5000 dilution of rabbit anti-TEP1, and rabbit anti-S7 as an internal control, in TBST blocking buffer overnight at 4 °C; For the detection of CSP expression, the membrane was incubated with rabbit anti-CSP-repeat, with rabbit anti-plasmodium hsp70 as an internal control. Membranes were then washed three times for 5 min in TBST and incubated with secondary anti-rabbit horseradish peroxidase (1:5000, Zhongshan Golden Bridge Biotechnology, Beijing, China) for 1 h at room temperature. After washing in TBST, the membrane was visualized using Western BLoT Chemiluminescence HRP Substrate (Takara Biotech Inc.). For comparative analysis between samples, densitometric analysis was performed using the software ImageJ. In vitro activation of mosquito hemocytes by oocysts On day 5, midguts from either CSP wt - or CSP mut -infected mosquitoes ( n = 20) with NOX5 knockdown or not were dissected and homogenized. The homogenate and hemocytes from un-infected mosquitoes ( n = 20) were incubated for 3 h at 28 °C, with medium containing antibiotics (including gentamicin, Sigma-Aldrich; penicillin/streptomycin/neomycin solution, Amphotericin B solution, Sangon, China). The medium containing antibiotics and uninfected midguts from mosquitoes were used as controls. After incubation, the incubation product was centrifuged at 500 × g for 30 s to remove mosquito tissue, and then the co-cultured hemocytes were collected with a centrifuge at 2000 × g for 5 min and smeared on coverslips pretreated with a poly-L-lysine solution. The immunofluorescence staining as described above was used to observe the nitration of hemocytes triggered by oocysts, and WGA (10 µg/mL, Invitrogen), which specifically marks mosquito hemocytes, was used to distinguish hemocytes from other mosquito cells. The mRNA levels of GNBP-B1 , Rel 1 , and TEP1 in hemocytes collected from naïve or from ds NOX5 mosquitoes were determined by quantitative real-time PCR analysis, as described above. Mosquito hemocyte depletion assay The day prior to CSP mut infection, naïve female mosquitoes (3–5 days old) were injected intrathoracically with either 69 nL of control liposomes or CLDs (Standard Macrophage Depletion Kit; Clodrosome ® + Encapsome ® ; Encapsula Nano Sciences, Brentwood, TN, USA) using a Nanoject II injector (Drummond Scientific Co.). As previously described [22] , 1:5 dilutions of liposomes and CLDs in 1 × PBS were used for the experiments. Following liposome injection, mosquitoes were infected with CSP mut parasites. The effect of clodronate liposomes on the depletion of mosquito hemocytes was determined by the expression of cell markers NimB2 (hemocytes), LRIM15 (granulocytes), and SCRB9 (oenocytoids) with real-time PCR as previously reported [26] . The change in oocyst melanization, the number of sporozoites, and relative expression of TEP1 were determined as described above. Statistical analysis All statistical analyses were performed using SPSS (IBM, Armonk, NY, USA). A Student’s t -test was used for two groups if the data were normally distributed to compare continuous variables, and if not, then the Mann–Whitney U test was used for comparisons among groups. Pairwise differences in normally distributed variables were compared using the one-way analysis of variance (ANOVA) for multiple comparisons. Significance was set at p < 0.05. Error bars represent the standard deviation (SD). Reporting summary Further information on research design is available in the Nature Research Reporting Summary linked to this article.